De novodesign of an RNA tile that self-assembles into a homo-octameric nanoprism Rational, de novo design of RNA nanostructures can potentially integrate a wide array of structural and functional diversities. Such nanostructures have great promises in biomedical applications. Despite impressive progress in this field, all RNA building blocks (or tiles) reported so far are not geometrically well defined. They are generally flexible and can only assemble into a mixture of complexes with different sizes. To achieve defined structures, multiple tiles with different sequences are needed. In this study, we design an RNA tile that can homo-oligomerize into a uniform RNA nanostructure. The designed RNA nanostructure is characterized by gel electrophoresis, atomic force microscopy and cryogenic electron microscopy imaging. We believe that development along this line would help RNA nanotechnology to reach the structural control that is currently associated with DNA nanotechnology. Self-assembled RNA nanostructures could potentially provide a platform to integrate a wide range of structural motifs and functionalities associated with RNA molecules, such as specific chemical binding [1] , catalysis capability [2] , gene regulation [3] and organizing proteins into large machineries [4] . They promise many technological applications, such as drug delivery [5] , [6] and arranging chemical reactions to produce useful chemicals [7] . Many exciting works have been reported recently along this line [8] , [9] . Often, natural RNA building blocks (also called as tiles or tectoRNAs) have been modified for such purposes [10] , [11] , [12] , [13] , [14] . Although convenient, this approach is limited to the structural elements of the natural building blocks. As a complementary approach, de novo design might offer higher versatility. Furthermore, such rational design also tests our knowledge about RNA and might allow us to build structures/functions that do not exist in nature but suit our needs. In biology, one basic building block can homo-oligomerize/polymerize into defined structures. For example, capsid proteins can self-assemble into well-defined viral capsids [15] and microtubulin can polymerize into long nanotubes [16] . In nanoengineering, DNA has been well explored for nanoconstruction and a range of well-behaved DNA building blocks (tiles) have been developed [17] , [18] . One single DNA tile can self-oligomerize/polymerize into nanocages, one-dimensional nanotubes, two-dimensional (2D) arrays and three-dimensional (3D) crystals [19] . In contrast, no RNA tile has been developed to have enough structural rigidity to homopolymerize/oligomerize into a defined large architecture. They will randomly associate into a mixture of complexes with different molecular weights. One potential way to overcome this problem is by using multiple tiles [10] , [11] , [12] , [13] , [14] , for example, using four tiles to form a heterotetramer. Can we rationally design RNA tiles that are structurally well defined so that they can polymerize/oligomerize into homo-oligomers with defined structures and molecular weights? Here, we report such a study: a de novo designed RNA tile that self-assembles into a homo-octameric cube. The self-assembly behaviour is characterized by gel electrophoresis, atomic force microscopy (AFM) and cryogenic electron microscopy (cryoEM) imaging. We believe that development along these lines would help RNA nanotechnology to reach the structural control that is currently associated with DNA nanotechnology. Molecular design The designed RNA tile is a two-stranded complex, R1–R2 ( Fig. 1a ). It contains three helical regions (P a , P b and P c ), two internal, single-stranded loops (L ab and L bc ) and two single-stranded tails (T a and T c ). This design integrates three important structural elements: a T-shaped junction (T-junction), a 90° bend and a sticky-end cohesion. First, the T-junction is adapted from a DNA T-junction [20] , [21] , [22] . The overall structure of a T-junction contains two duplexes with one duplex perpendicularly (90°) stacking onto the major groove of the second one. It forms when a single-stranded tail (5–6 bases long) of a duplex hybridizes with a single-stranded loop of another duplex ( Fig. 1b ). We hypothesize that such a T-junction architecture will be equally compatible with RNA (A-form duplex) and DNA (B-form duplex) [23] , [24] , [25] . Here T a tail–L ab loop base pairing among the tiles will cause the tiles to tetramerize and form a square ( Fig. 1c ). Note that each side of the square is two helical turns, or 22 base pairs (bp) long. Second, the 90° bend is taken from a naturally existing RNA element present in the internal ribosome entry site (IRES) of the hepatitis C virus (HCV) RNA genome [26] . Helix P b is chosen to be 7 bp (~¾ helical turn) long so that the 90° bend would make the P c domain to protrude out of the square plane by 90° ( Fig. 1c ). Third, tail T c is a self-complementary sticky end. Tiles can homo-dimerize through sticky-end (T c ) cohesion. Sticky-end (T c ) cohesion will produce a long, continuous duplex that is 6+4+6=16 bp (1.5 turns) long. This length will present the two square planes to face each other. Conceptually, we think that the tiles first form homo-tetramers (squares) via T-junctions and the squares further homo-dimerize via sticky-end (T c ) cohesion. Thus, the final RNA complex will be homo-octamer of the tiles, cube-like structures. However, the assembly in solution probably is more like a cooperative assembly instead of a sequential assembly. 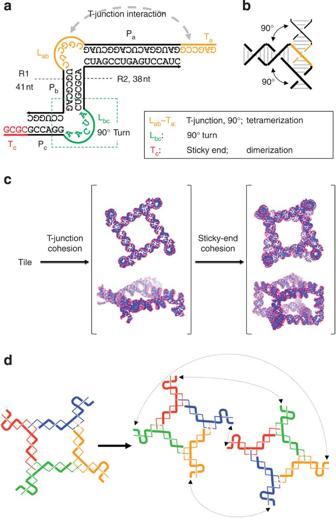Figure 1: Self-assembly of ade novodesigned RNA tile into a homo-octameric prism. (a) Sequence and secondary structure of the design, two-stranded RNA tile (R1–R2). All structural elements (three duplex regions Pa, Pband Pc; two tails Taand Tc; two internal bulges loops Laband Lbc) are indicated. Note that Ta(yellow) and Lab(yellow) are complementary to each other and Tc(red) is self-complementary. (b) A detailed scheme of a T-junction structure formed by hybridization between a Tatail and Labloop. Both are coloured yellow. The black and yellow lines represent the RNA backbones and the short grey lines represent base pairs. (c) Self-oligomerization of the RNA tile. The tile can tetramerize into tetrameric square via T-junction formation (Ta–Labhetero-hybridization) and dimerize via sticky-end cohesion (Tc–Tchybridization). The two types of interactions together lead to the formation of an octameric nanoprism. For both the square and prism, a top view and a near side view are shown. The structural models were prepared with a computer program Coot. (d) A 2D diagram showing the connectivity of the tiles. Each tile contains two strands represented by a thick line and a thin line, which share the same colour. Figure 1: Self-assembly of a de novo designed RNA tile into a homo-octameric prism. ( a ) Sequence and secondary structure of the design, two-stranded RNA tile (R1–R2). All structural elements (three duplex regions P a , P b and P c ; two tails T a and T c ; two internal bulges loops L ab and L bc ) are indicated. Note that T a (yellow) and L ab (yellow) are complementary to each other and T c (red) is self-complementary. ( b ) A detailed scheme of a T-junction structure formed by hybridization between a T a tail and L ab loop. Both are coloured yellow. The black and yellow lines represent the RNA backbones and the short grey lines represent base pairs. ( c ) Self-oligomerization of the RNA tile. The tile can tetramerize into tetrameric square via T-junction formation (T a –L ab hetero-hybridization) and dimerize via sticky-end cohesion (T c –T c hybridization). The two types of interactions together lead to the formation of an octameric nanoprism. For both the square and prism, a top view and a near side view are shown. The structural models were prepared with a computer program Coot. ( d ) A 2D diagram showing the connectivity of the tiles. Each tile contains two strands represented by a thick line and a thin line, which share the same colour. Full size image Electrophoretic study RNA assembly was carried out by following the previously reported method [14] . Two-component strands at equal molar ratio were mixed in an Mg 2+ -containing, aqueous buffer and slowly cooled from 80 °C to 22 °C in 2 h. The assembly mixture was first analysed by native polyacrylamide gel electrophoresis (PAGE). 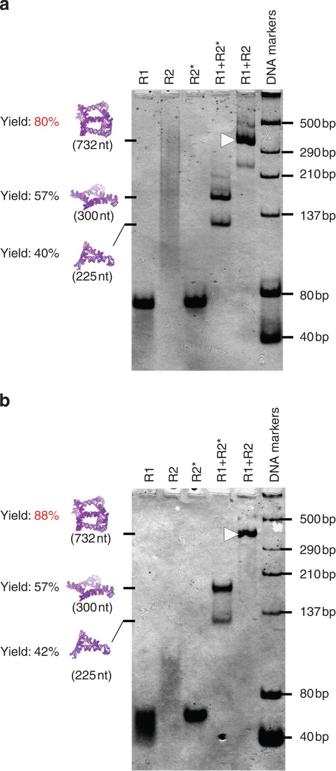Figure 2: Native PAGE of the self-assembly of the RNA prism. The 6% PAGE was performed at two different temperatures: (a) 22 °C and (b) 50 °C. R2* has the same sequence as R2 except the Tctail is removed. Thus R1–R2* complex can interact with each other only via T-junction to form tetrameric squares, but not prisms. On the far right of each gel images are a series of DNA duplex size markers. For each gel, the sample composition in each lane and the chemical identity of each band are indicated above and beside the gel images, respectively. The white arrowheads indicate the homo-octameric prisms. Note that the assembly yields of the targeted prism, square and triangle are estimated by ImageJ32based on the band intensities. Figure 2 shows the experimental result. The left two lanes are the individual component RNA strands. R1 sample appears as a sharp band, whose mobility suggests that R1 self-associates into dimers. R2 self-oligomerizes into a mixture, which smears out in the gel. The abnormal association behaviour of R2 can be partly attributed to the T c tail. When this tail is removed (R2*), it appears as a sharp, strong band just like R1. Without the T c tail, the blunt tile (R1−R2*) is supposed to form a planar tetramer via T-junction association; however, it cannot further dimerize into cube-like structure. This is consistent with the PAGE data. In addition to the main square product (57%), significant of triangle (40%) and trace amount of pentagon also exist. With the T c tail, the tile self-associates into a cube-like octamer (dimer of tetramer) that shows as a dominant (80%), sharp band in the gel. Two weak bands appear either above or below the cube. There are two interesting phenomena in the native PAGE. First, the yield (80%) of cube-like octamer is higher than that (57%) of square tetramer. The sticky-end (T c ) cohesion influences the T-junction association. Such a synergistic assembly behaviour suggests that the final cube-like structure is not assembled from the pre-assembled square structure. Instead, the cube-like structure is simultaneously assembled cooperatively from the tiles via T-junction formation and sticky-end (T c ) cohesion. Second, those undesired by-products in the lanes of R1+R2 and R1−R2* are not as stable as the desired RNA complexes. The bands of those by-products significantly decrease while the bands of the desired RNA complexes remain the same, indicating that the desired structures are energetically more stable than other by-products. Figure 2: Native PAGE of the self-assembly of the RNA prism. The 6% PAGE was performed at two different temperatures: ( a ) 22 °C and ( b ) 50 °C. R2* has the same sequence as R2 except the T c tail is removed. Thus R1–R2* complex can interact with each other only via T-junction to form tetrameric squares, but not prisms. On the far right of each gel images are a series of DNA duplex size markers. For each gel, the sample composition in each lane and the chemical identity of each band are indicated above and beside the gel images, respectively. The white arrowheads indicate the homo-octameric prisms. Note that the assembly yields of the targeted prism, square and triangle are estimated by ImageJ [32] based on the band intensities. Full size image AFM imaging We have further applied AFM to examine the geometric structures of the assembled RNA complexes ( Fig. 3 ). For blunt-ended sample, R1+R2*, the individual particles (height: 1.2 nm) are randomly distributed on the surfaces. At high magnification, different geometries can be clearly resolved. Statistically, there are ~37% triangle and~59% square, consistent with the observation by native PAGE. For the sample with sticky ends, R1+R2, the dominating particles exhibit a rectangle shape (14 × 12 nm). The particle height (2.8 nm) strongly suggests that they are not 2D, planar, 2D planar structures. Instead, they are the collapsed 3D structures. Both their shape and height indicate that they are the designed cube-like structures. Note that the apparent height (2.8 nm) is much less than the expected 7 nm. It is likely due to that the RNA cages collapse on the AMF substrate because of the strong electrostatic interaction between the RNA molecules and the substrate (mica) surface, and the dehydration required for imaging in air. 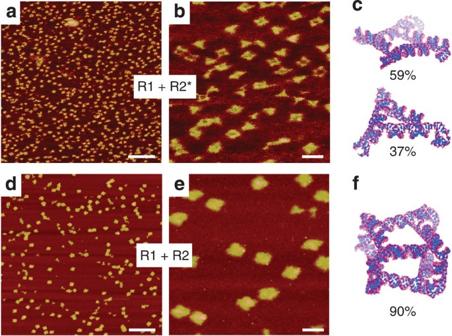Figure 3: AFM characterization of RNA complexes. (a) An AFM image of the assembly products of R1+R2*, (b) its close-up view and (c) structural models of the two main products: square and triangle. (d) An AFM image of assembly mixture of R1+R2, (e) its close-up view and (f) the structural model of the prism. Structural models are prepared with Coot. Scale bar, 100 nm (a,d); 20 nm (b,e). Figure 3: AFM characterization of RNA complexes. ( a ) An AFM image of the assembly products of R1+R2*, ( b ) its close-up view and ( c ) structural models of the two main products: square and triangle. ( d ) An AFM image of assembly mixture of R1+R2, ( e ) its close-up view and ( f ) the structural model of the prism. Structural models are prepared with Coot. Scale bar, 100 nm ( a , d ); 20 nm ( b , e ). Full size image Cryogenic electron microscopy To directly reveal the native 3D structure of the assembled RNA complex, we have imaged the RNA sample by cryoEM ( Fig. 4 ) [27] . In raw cryoEM images, the individual particles can be easily identified (indicated by white boxes). Their shapes resemble the expected 2D projections of the designed prism. With the observed individual RNA particles, the original 3D structures of the RNA complexes are reconstructed by a single-particle 3D reconstruction technique [28] , [29] , which results in a structural model of tetragonal prism at a resolution of 2.1 nm. One step further, we made two pair comparisons between the computed 2D projections of the reconstructed model with individual raw particles observed in cryEM images ( Fig. 4d ) and with class average of raw particles with similar views ( Fig. 5 ). Clear similarities observed in those comparisons further verified the reconstructed model. 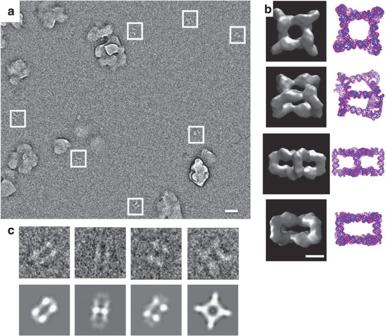Figure 4: CryoEM of the self-assembled homo-octameric RNA nanoprism. (a) A raw cryoEM image of the RNA complex. Each white box indicates an individual RNA complex. Large irregular structures are ice crystals. Scale bar, 25 nm. (b) The reconstructed structural model of the RNA complex viewed from different orientations and the corresponding views of the simulated model. Scale bar, 5 nm. (c) Pairwise comparison between individual raw particles and computer-generated 2D projections of the reconstructed 3D structural model in similar orientations. Figure 4: CryoEM of the self-assembled homo-octameric RNA nanoprism. ( a ) A raw cryoEM image of the RNA complex. Each white box indicates an individual RNA complex. Large irregular structures are ice crystals. Scale bar, 25 nm. ( b ) The reconstructed structural model of the RNA complex viewed from different orientations and the corresponding views of the simulated model. Scale bar, 5 nm. ( c ) Pairwise comparison between individual raw particles and computer-generated 2D projections of the reconstructed 3D structural model in similar orientations. 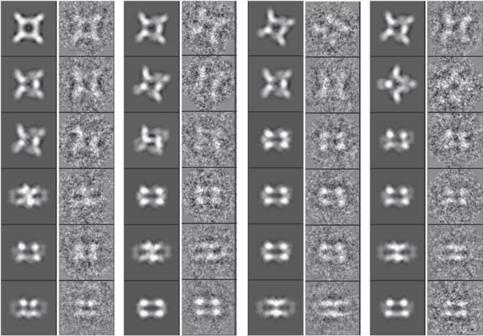Figure 5: Validating the reconstructed prism structure. Pairwise comparison between class averages of the raw images of individual particles and the corresponding 2D projections of the reconstructed 3D structural model in similar orientations. Full size image Figure 5: Validating the reconstructed prism structure. Pairwise comparison between class averages of the raw images of individual particles and the corresponding 2D projections of the reconstructed 3D structural model in similar orientations. Full size image Co-transcriptional assembly The RNA self-assembly in this study is a robust process. It readily processes even though the RNAs are not pure and there are many other molecules, including RNA polymerase, DNA templates and other related RNA molecules. We have performed one control experiment. The DNA templates of the two-component RNA strands are mixed. On addition of RNA polymerase, co-transcription produces the two RNA strands. Without any purification, the transcription mixture is thermally annealed and analysed by native PAGE ( Fig. 6 ). A strong band appears at the position of the target prism complex although the assembly yield is not clear. Thus, RNA purification after transcription is not a necessary process as also demonstrated by other studies [24] , [30] . It overcomes one of the problems that are faced by self-assembly of RNA nanostructures in cells, where RNA purification is not possible. 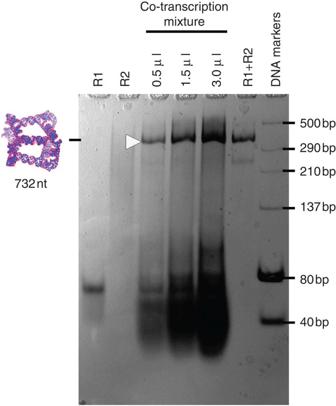Figure 6: Self-assembly of the RNA prism from transcription mixture. The middle three lanes are RNA samples directly annealed from co-transcribed raw RNAs without any purification or fraction. The loading amounts are different. Sample R1+R2 is a size marker, which is assembled from purified RNAs. Figure 6: Self-assembly of the RNA prism from transcription mixture. The middle three lanes are RNA samples directly annealed from co-transcribed raw RNAs without any purification or fraction. The loading amounts are different. Sample R1+R2 is a size marker, which is assembled from purified RNAs. Full size image We have successfully integrated a naturally existing RNA structural building block (90° bend) and a non-natural, artificially designed structural building block (T-junction) to design an RNA tile, which can readily homo-oligomerize into a predesigned, large architecture. It is a great challenge to design an RNA tile that can homo-oligomerize into a defined nanostructure. To the best of our knowledge, there is only one report in the literature, where an RNA duplex with an internal loop (a natural-existing 90° bend) self-tetramerizes into a square [31] . Here we expand the design principle to achieve higher structural complexity along this direction. Besides addressing the fundamental challenge in programmed RNA self-assembly, we believe that such a study will increase our capability of rationally designing RNA nanostructures [33] , [34] to meet the needs of potential applications such as siRNA delivery [5] , [6] and construction of in vivo RNA machineries [4] . In addition, we have observed a surprising but interesting phenomenon. There is a synergistic effect between different inter-tile interactions (T-linkage association and sticky-end cohesion). It promotes the assembly of one particular structure among many possible structures. Such an effect might be general in molecular self-assembly; which, however, needs to be further tested. Oligonucleotides All DNA strands were purchased from IDT, Inc. and purified by 20% denaturing PAGE. T7 promoter sequences are underlined. R1: 5′-GAG CCG GAU GGA CUC AGG CUA GCG GCU CUG CGC AGC CUG GC-3′. R2: 5′-GCG CGC CAG GAA CUA CUG CGC ACU AGC CUG AGU CCA UC-3′. R2*: 5′- GCC AGG AAC UAC UGC GCA CUA GCC UGA GUC CAU C-3′. DNA template strands for R1: 5′- TTC TAA TAC GAC TCA CTA TA G AGC CGG ATG GAC TCA GGC TAG CGG CTC TGC GCA GCC TGG C-3′; 5′-GCC AGG CTG CGC AGA GCC GCT AGC CTG AGT CCA TCC GGC TC T ATA GTG AGT CGT ATT AGA A -3′. DNA template for R2: 5′- TTC TAA TAC GAC TCA CTA TA G CGC GCC AGG AAC TAC TGC GCA CTA GCC TGA GTC CAT C-3′; 5′-GAT GGA CTC AGG CTA GTG CGC AGT AGT TCC TGG CGC GC T ATA GTG AGT CGT ATT AGA A -3′. DNA template for R2*: 5′- TTC TAA TAC GAC TCA CTA TA G CCA GGA ACT ACT GCG CAC TAG CCT GAG TCC ATC-3′; 5′-GAT GGA CTC AGG CTA GTG CGC AGT AGT TCC TGG C TA TAG TGA GTC GTA TTA GAA -3′. RNA preparation All RNA molecules are synthesized by in vitro transcription with T7 RNA polymerase (the AmpliScribe T7-Flash transcription kit; Epicenter, Inc.) from corresponding DNA templates by following the manufacturer-recommended protocol, and then purified using the 20% denaturing PAGE. Formation of RNA prisms Two-component RNA strands (R1+R2 or R1+R2*) at 2 μM were combined in TAE/Mg 2+ buffer and incubated at 80 °C for 5 min, 65 °C for 15 min, 50 °C for 30 min and 22 °C for 30 min. TAE/Mg 2+ buffer contained 40 mM Tris base (pH 8.0), 20 mM acetic acid, 2 mM EDTA and 12.5 mM magnesium acetate. Denaturing PAGE The 20% denaturing PAGE gel was prepared with 19:1 acrylamide/bisacrylamide gel, 8 M urea and TBE buffer (89 mM Tris base (pH=8.0), 89 mM boric acid and 2 mM EDTA). The gel was run at 55 °C for 2 h at 650 V on Hoefer SE 600 electrophoresis system and then stained with ethidium bromide (Sigma). The major band was cut under ultraviolet light and eluted out. Native PAGE The 6% native PAGE gel is prepared with 19:1 acrylamide/biacrylamide gel and TAE/Mg 2+ buffer. The gel was run at 22 or 50 °C, stained with Stains-All (Sigma) and scanned by an HP scanner (Scanjet 4070 Photosmart). For 22 °C gel, samples were directly used after annealing. For 55 °C gel, the sample was cooled to room temperature and incubated at 50 °C for 1 h before electrophoresis. AFM imaging A drop of 4 μl annealed RNA solution was deposited onto freshly cleaved mica substrate and incubated for 1 min. Then the mica surface was washed by 30 μl 2 mM Mg 2+ aqueous solution to remove excess salts and any unbounded RNA complexes. AFM imaging was carried out on a Bruker MultiMode 8 AFM at SCANASYST-AIR mode with ScanAsyst-Air Silicon Nitride probe (Bruker). Computationally building the 3D model of the prism We started to build the 3D model from building the tile by joining A-form RNA duplexes with T-junction loop and 5-nt loop that generated 90° turn. T-junction loop was adapted from a DNA T-junction [19] , [20] , [21] and generated in computer software Win COOT to ensure the T-shape. To manually connect the 6-nt loop with the duplex (indicated as P a in Fig. 1a ), we manipulated P a to ensure that base C in loop L ab was close to base G on P a and that base A on P b was close to base C on P a so that they could be joined together. The angle between P a and P b was controlled to be about 90°. The length of P b was determined to be 7 bp to ensure duplex P c would rotate 90° to be perpendicular to the RNA square. The 90° turn, 5-nt loop L bc was extracted from the crystal structure (PDB_ID: 3P59) in the RCSB PDB database. The length of duplex P c was subjected to change and determined at the last. We first assembled the RNA square by inserting the T a tail of one tile into the L ab loop of another tile (T-junction interaction). As formed RNA square had four duplexes perpendicularly sticking out of the plane and facing the same side. By merging two such squares, we were able to determine that P c could be 6-bp long and T c could be 4 nt. We would like to point out that the such-generated 3D model is not energy-minimized 3D structure; instead, it serves as a convenient visual illustration. CryoEM imaging Three microlitres of solution (RNA concentration: 3 μM) was deposited on the Quantifoil grid (Electron Microscopy Sciences, Q250-CR2-400). The grid was blotted with two pieces of filter paper (Whatman, 1001-055) and immediately flash frozen by liquid nitrogen-cooled liquid ethane. Images were taken on FEI CM200 TEM with accelerating voltage of 200 kV under low-dose condition to minimize radiation damages to the samples. To enhance the image contrast, under-focus in the range of 2–4 μm were used to record the images by films. Single-particle reconstruction The single-particle reconstruction was carried out using computer software EMAN 2 (ref. 28 ). Totally, 400 particles were selected to go through reconstruction process using EMAN2 reconstruction package following the standard protocol. All the data were processed following EMAN2 reconstruction tutorial using the workflow interface, provided via Wiki at: http://blake.bcm.edu . A general summary of the steps include: import and pre-process micrographs; picking particles; CTF determination; remove bad particles and build particle sets; make 2D reference-free class averages; build an initial 3D model; 3D high-resolution refinement; evaluate the resolution of a 3D map. About 200 randomly selected particles were used to build 12 class averages, which were used to generate initial models. The initial orientations of individual particles were randomly assigned within the corresponding asymmetric units of the D4 symmetry for the Nanoprism. With a C4 symmetry (a lower symmetry), a similar structural map was obtained. Totally, over 400 particles were used for the 3D refinements of the Nanoprism. The refinement was carried out with a 2° angle interval. A projection-matching algorithm was applied for the determination of the centre and orientation of the raw particles in the iterative refinement for the prism. The corresponding symmetry was imposed during the reconstruction. After the refinement, class averages of the raw particles and 2D projections of the 3D model were generated in two files but paired in order. The comparisons presented were manually selected to show the distinct and comprehensive orientations. The resolution of the resulted structural density map was determined to be at 2.1 nm, with the Fourier shell correlation (0.5 threshold criterion). Final reconstruction results were visualized by UCSF Chimera software. How to cite this article: Yu, J. et al. De novo design of an RNA tile that self-assembles into a homo-octameric nanoprism. Nat. Commun. 6:5724 doi: 10.1038/ncomms6724 (2015).